Neovenatorid theropods are apex predators in the Late Cretaceous of North America Allosauroid theropods were a diverse and widespread radiation of Jurassic–Cretaceous megapredators. Achieving some of the largest body sizes among theropod dinosaurs, these colossal hunters dominated terrestrial ecosystems until a faunal turnover redefined apex predator guild occupancy during the final 20 million years of the Cretaceous. Here we describe a giant new species of allosauroid – Siats meekerorum gen. et sp. nov. – providing the first evidence for the cosmopolitan clade Neovenatoridae in North America. Siats is the youngest allosauroid yet discovered from the continent and demonstrates that the clade endured there into the Late Cretaceous. The discovery provides new evidence for ecologic sympatry of large allosauroids and small-bodied tyrannosauroids. These data support the hypothesis that extinction of Allosauroidea in terrestrial ecosystems of North America permitted ecological release of tyrannosauroids, which went on to dominate end-Cretaceous food webs. Over a century of collection efforts have rendered Late Jurassic and latest Cretaceous (Campano-Maastrichtian) terrestrial ecosystems in western North America among most densely sampled and comprehensively understood dinosaur faunas in the world [1] , [2] , [3] . These distinct windows into North American dinosaur evolution stand in marked contrast to each other in taxonomic content, degree of endemism and body mass composition, and together bracket a dramatic faunal reorganization of apex predatory guilds on the continent [4] . Whereas Late Jurassic assemblages contain a diverse community of medium to large-bodied predators including piatnitzkysaurids, megalosaurids, allosaurids, ceratosaurids and basal tyrannosauroids [5] , apex predator guilds in the latest Cretaceous were taxonomically depauperate, being dominated exclusively by one to three tyrannosaurid species with subsidiary roles occupied by a variety of maniraptoran clades [6] , [7] . Characterizing the pattern and tempo of this restructuring is paramount to understanding diversity, biogeography, extinction and replacement between well-sampled North American faunas [8] , and carries significant implications for spatiotemporal patterns of faunal composition on a global scale [1] , [9] , [10] . However, poor sampling of the apex predator niche in the mid-Cretaceous is a persistent and wide-ranging problem [11] . The paucity of pre-Campanian data on top predators of North America is particularly extreme, with only a single taxon, Acrocanthosaurus [12] , described from the first 70 million years of the Cretaceous. Such sampling biases have led to the hypothesis that predator assemblages during this interval were depauperate and homogeneous across the continent [13] and have obscured the timing of major ecological events such as the ascension of tyrannosauroids to top predator roles [14] . Whether this turnover was related to out competition of endemic allosauroids or rather, release from competitive exclusion via regional extinction events as has been suggested for other Laurasian landmasses [14] , [15] and earlier Mesozoic radiations [16] , [17] remains unclear. Here we document the previously unrecognized presence of neovenatorid allosauroids as top predators in what are now known to be taxonomically distinct mid-Cretaceous faunas of North America. This finding provides new data on the pace and characterization of guild restructuring and indicates that the complexity of apex predator dynamics and diversity in the region is underappreciated. In particular, our finding, coupled with sympatric association of diminutive tyrannosaur species from the same rock units, suggests that occupation by carcharodontosaurians likely excluded tyrannosauroids from top predator niches through, at minimum, the early Late Cretaceous of North America. Systematic palaeontology Theropoda Marsh 1881 Allosauroidea Marsh 1878 Neovenatoridae Benson, Carrano, Brusatte 2009 Megaraptora Benson, Carrano, Brusatte 2009 Siats meekerorum gen. et sp. nov. Holotype. FMNH (Field Museum of Natural History) PR 2716, partial postcranial skeleton of immature individual including portions of the axial column, pelvic girdle and hind limb ( Fig. 1 ). Immaturity of the holotype is evident from lack of neurocentral fusion across the axial series except in distal caudals. 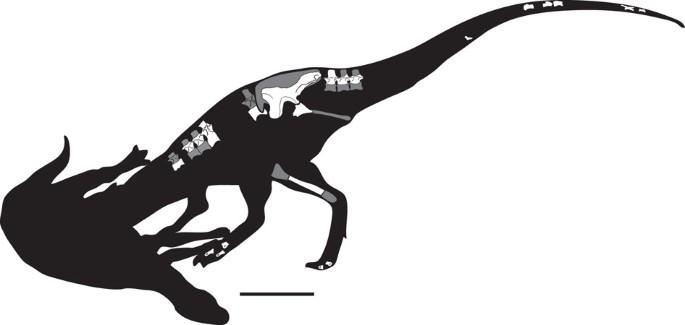Figure 1: Skeletal reconstruction ofS. meekerorumshown preying onEolambia caroljonesi. Preserved elements of the axial and appendicular skeleton shown in white; missing portions outlined in grey. Scale bar, 1 m. Select measurements are provided in Table 1 . Figure 1: Skeletal reconstruction of S. meekerorum shown preying on Eolambia caroljonesi . Preserved elements of the axial and appendicular skeleton shown in white; missing portions outlined in grey. Scale bar, 1 m. Full size image Table 1 Measurements of S. meekerorum holotype FMNH PR 2716. Full size table Referred specimen. FMNH PR 3059, a mid-caudal neural arch and chevron, a pedal phalanx and several indeterminate bone fragments. Etymology. Siats , a predatory, man-eating monster from legends of the Ute native tribe of Utah (occasionally spelled as See-atch), and meekerorum , honouring the Meeker family for their endowment in support of early career palaeontologists at the Field Museum. Locality and horizon. Mussentuchit Member, ~98 Ma [18] , Upper Cretaceous (Cenomanian) Cedar Mountain Formation, ~10 m below the base of the Dakota Formation; Emery County, Utah, USA (exact coordinates on file). The holotype was recovered disarticulated, yet associated, from a paucispecific bone bed also containing small theropod and abundant microvertebrate remains. Diagnosis. Large-bodied allosauroid exhibiting craniocaudally expanded centrodiapophyseal laminae yet lacking well-developed infradiapophyseal fossae on proximal caudals (autapomorphy) ( Fig. 2i ); craniocaudal elongation of craniodorsal centra ( Fig. 2a ); abbreviated, transversely broad neural spines on dorsal vertebrae (neural spine height ~50% maximum height of centrum) ( Fig. 2d,e ); transversely flattened, axially concave ventral surface yielding subtriangular cross-section on distal caudal vertebrae (autapomorphy) ( Fig. 2j,k ); transversely concave acetabular rim of iliac pubic peduncle (autapomorphy) ( Fig. 3a ); truncated lateral brevis shelf with notched caudal end (autapomorphy) ( Fig. 3a ); brevis fossa with subparallel mediolateral margins; supraacetabular crest truncated above midpoint of acetabular rim ( Fig. 3a ). 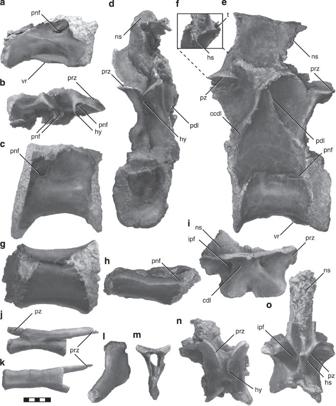Figure 2: Select axial elements of the holotype ofS. meekerorum. (a) Cranial dorsal centrum in right lateral view; (b) cranial dorsal prezygapophyses in oblique rostral view, showing prezygapophyseal pneumaticity; (c) caudal dorsal centrum in left lateral view; cranial (possible fifth) dorsal vertebra, in (d) cranial and (e) right lateral views, (f) inset showing lateral tab on postzygapophysis; probable sacral centrum in (g) ventral and (h) right lateral views; (i) cranial (third or fourth) caudal neural arch in right lateral view; distal caudal vertebra in (j) right lateral and (k) ventral views; cranial chevron in (l) right lateral and (m) caudal views; (n) cranial caudal neural arch in cranial view, showing hypantrum; (o) cranial caudal neural arch in caudal view. Scale bar, 5 cm. ccdl, caudal centrodiapophyseal lamina; cdl, centrodiapophyseal lamina; hs, hyposphen; hy, hypantrum; ipf, infrapostzygapophyseal fossa; ns, neural spine; pdl, paradiapophyseal lamina; pnf, pneumatic foramina; prz, prezygapophysis; pz, postzygapophysis; t, tab on postzygapophysis; vr, ventral ridge. Figure 2: Select axial elements of the holotype of S. meekerorum. ( a ) Cranial dorsal centrum in right lateral view; ( b ) cranial dorsal prezygapophyses in oblique rostral view, showing prezygapophyseal pneumaticity; ( c ) caudal dorsal centrum in left lateral view; cranial (possible fifth) dorsal vertebra, in ( d ) cranial and ( e ) right lateral views, ( f ) inset showing lateral tab on postzygapophysis; probable sacral centrum in ( g ) ventral and ( h ) right lateral views; ( i ) cranial (third or fourth) caudal neural arch in right lateral view; distal caudal vertebra in ( j ) right lateral and ( k ) ventral views; cranial chevron in ( l ) right lateral and ( m ) caudal views; ( n ) cranial caudal neural arch in cranial view, showing hypantrum; ( o ) cranial caudal neural arch in caudal view. Scale bar, 5 cm. ccdl, caudal centrodiapophyseal lamina; cdl, centrodiapophyseal lamina; hs, hyposphen; hy, hypantrum; ipf, infrapostzygapophyseal fossa; ns, neural spine; pdl, paradiapophyseal lamina; pnf, pneumatic foramina; prz, prezygapophysis; pz, postzygapophysis; t, tab on postzygapophysis; vr, ventral ridge. 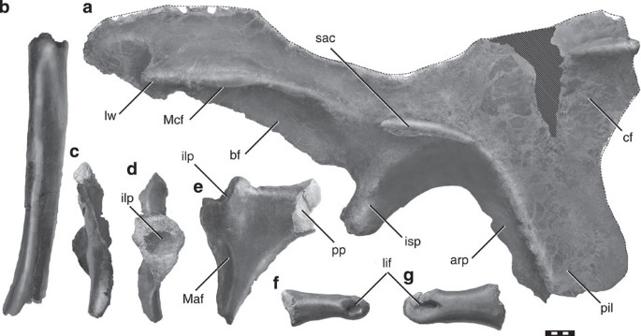Figure 3: Select pelvic and hindlimb elements of the holotype ofS. meekerorum. (a) Right ilium in lateral view; (b) fibula in lateral view; right ischium in (c) ventral, (d) proximal and (e) lateral views; (f) pedal phalanx III-2 in lateral view; (g) right pedal phalanx II-1 in medial view. Scale bar: 5 cm. arp, acetabular rim of pubic peduncle of ilium; bf, brevis fossa; cf, cuppedicus fossa; ilp, iliac peduncle of ischium; isp, ischial peduncle of ilium; lif, ligament fossa; lw, lateral wall of brevis fossa; Maf, M. adductor femoris scar on ischium; Mcf, M. caudofemoralis origin; pil, pubic peduncle of ilium; pp, pubic peduncle of ischium. Full size image Figure 3: Select pelvic and hindlimb elements of the holotype of S. meekerorum. ( a ) Right ilium in lateral view; ( b ) fibula in lateral view; right ischium in ( c ) ventral, ( d ) proximal and ( e ) lateral views; ( f ) pedal phalanx III-2 in lateral view; ( g ) right pedal phalanx II-1 in medial view. Scale bar: 5 cm. arp, acetabular rim of pubic peduncle of ilium; bf, brevis fossa; cf, cuppedicus fossa; ilp, iliac peduncle of ischium; isp, ischial peduncle of ilium; lif, ligament fossa; lw, lateral wall of brevis fossa; Maf, M. adductor femoris scar on ischium; Mcf, M. caudofemoralis origin; pil, pubic peduncle of ilium; pp, pubic peduncle of ischium. Full size image Description and comparisons With the exception of several, potentially referable isolated teeth, no cranial materials are known for Siats . Parts of five dorsal and up to 13 caudal vertebrae were recovered ( Fig. 1 ) with other fragmentary elements possibly pertaining to the sacrum or cervical series. Presacral vertebrae exhibit camellate pneumaticity and pneumatic foramina are present on all preserved presacral centra. All recovered vertebral neural arches are unfused, with the exception of distal-most caudal vertebrae, indicating that the holotype represents a skeletally immature individual ( Fig. 2 ). Recovered portions of the dorsal series include an isolated cranial dorsal centrum ( Fig. 2a ); two fragmentary dorsal neural arches ( Fig. 2b ); a nearly complete, probable fifth cranial dorsal vertebra ( Fig. 2d,e ) missing its transverse processes and left postzygapophysis; an isolated caudal dorsal centrum ( Fig. 2c ); and several additional fragments including multiple isolated pre- and postzygapophyses. All dorsal centra are platycoelous and bear dorsally directed, slit-like pneumatopores ( Fig. 2c,e ). The cranial-most centrum is transversely constricted and bears a ventral ridge as in Neovenator and Aerosteon [19] . Rostrally, this ridge appears to deepen into a knob that may be the base of a blunt hypapophysis ( Fig. 2a ). In contrast to Neovenator , the cranial dorsal centra are markedly elongate (more than twice as long as tall) ( Fig. 2a ). Two partial neural arches from cranial dorsals exhibit pneumatic prezygapophyses ( Fig. 2b ) bearing transversely expanded (as in Ilokelesia [20] ) and quadrangular hypantra similar to the condition observed in Aerosteon . Articular faces on the cranial-most dorsal vertebrae are wider than tall (width to height ratios 1.13–1.31). The probable fifth dorsal exhibits a low but distinct ventral ridge ( Fig. 2e ), articular faces that are taller than wide (130%), flange-like lateral extensions of the postzygapophyses as in Neovenator and Aerosteon [19] ( Fig. 2e,f ), and a hypertrophied caudal centrodiapophyseal lamina. In contrast to the deep hypaxial portion of the arch, the neuralspine is compact (less than the height of the centrum; Fig. 2d,e ), and transversely broad at its base, unlike the tall, buttressed dorsal neural spines of Acrocanthosaurus and other carcharodontosaurids. Dorsal hyposphens are distinct and alariform as in other carcharodontosaurids [19] , yet flare ventrolaterally at their distal-most extent ( Fig. 2e,f ). A dorsoventrally flattened, ventrally rounded centrum exhibiting interior camellate pneumaticity may represent a sacral ( Fig. 2g,h ). A series of three rostral caudal neural arches are variably preserved and likely represent the first through third or second through fourth caudals ( Figs 1 and 2i,n,o ). Pre- and postzygapophyses are spaced close to the midline ( Fig. 2n,o ), in contrast to Neovenator, in which they flare laterally [21] . Their articular facets are flexed and curve ventromedially with those of the postzygapophyses meeting ventrally to form hyposphen–hypantrum articulations ( Fig. 2n,o ) as in Sinraptor and some allosauroids [22] , yet not Allosaurus [23] . Short transverse processes are fan-shaped, backswept and project horizontally from the neural arch. They are braced by a single, craniocaudally wide centrodiapophyseal lamina ( Fig. 2i ), which is excavated by deep infrapre- and infrapostzygapophyseal fossae ( Fig. 2i,o ); presence of these diagnostic fossae permit referral of FMNH PR 3059 to Siats . Well-developed neural arch fossae are observed in the rostral caudal vertebrae of Aerosteon and Megaraptor , and have been interpreted as a synapomorphy of these taxa [19] , but absence of a well-developed infradiapophyseal fossa is autapomorphic to Siats ( Fig. 2i ). Distal caudal vertebrae are amphicoelous to platycoelous, and have centra with a unique subtriangular cross-section at midlength and wide, transversely flat and axially concave ventral surfaces ( Fig. 2j,k ). They lack a midline groove such as occurs in other allosauroids including Allosaurus [24] , Neovenator [21] and Mapusaurus [25] , and bear moderately elongated prezygapophyses. A mid-caudal chevron is transversely flattened and distally expanded and its proximal articulations are connected forming a roof over the haemal canal ( Fig. 2l,m ). Preserved pelvic elements include a partial right ilium ( Fig. 3a ) and proximal portions of the right and left ischium ( Fig. 3c-e ). Most of the preacetabular wing and mid-blade of the ilium are not preserved. The base of the preacetabular wing bears a lateral flange that defines a deep cuppedicus fossa as found in megaraptoran allosaurids and tyrannosauroids ( Fig. 3a ). Poor preservation including crushing and fragmentation have flattened the ilium and everted the medial wall of the cuppedicus fossa and cranial pubic peduncle, obscuring their original morphology. A pronounced supracetabular crest terminates as a dorsocaudally inclined, caudally thickened and truncated flange rostral to the level of the ischial peduncle ( Fig. 3a ). The postacetabular wing bears a distally truncated lateral wall to the M. caudofemoralis brevis shelf, as in Megalosaurus [22] (BMNH R1100; Natural History Museum (formerly British Museum of Natural History) and Eustreptospondylus [26] , and possibly Torvosaurus [19] , yet is distinctive in exhibiting a cranially concave terminus ( Fig. 3a ). The lateral wall of the brevis shelf is also reduced dorsoventrally, exposing the ventral aspect of the medial shelf in lateral view. Distally, the ventral margin of the lateral shelf bears a bulbous expansion for origination of the M. caudofemoralis brevis ( Fig. 3a ) as in Neovenator (NHMUK R 10001). The brevis fossa is deep with subparallel medial and lateral margins as in metriacanthosaurids, yet lacks the pneumatopores present on Mapusaurus [25] , Aerosteon [26] and probably Giganotosaurus [27] (MUCPv-Ch-1)(Museo de la Universidad Nacional de Comahue – El Chocón collection) (see Supplementary Note 1 and Supplementary Data 1 ). The proximal ischium is plate-like and tapers rapidly to a gracile shaft. Although the shape of the obturator process cannot be determined, an obturator foramen was clearly absent ( Fig. 3c ). The acetabular margin is relatively straight in lateral view ( Fig. 3e ), with a dorsally beveled surface that is convex laterally and concave medially as in Neovenator . A deep furrow for the M. adductor femoris 2 excavates the caudolateral aspect of the proximal ischium ( Fig. 3e ). This furrow demarcates a rugose crest confluent with the caudal aspect of the ischial shaft as in Sinraptor [23] and Mapusaurus [25] . As in other carcharodontosaurians [19] , the ilio–ischial articulation is formed as a peg and socket joint ( Fig. 3d,e ). A long section (~460 mm) of the transversely compressed fibular shaft distal to the M. iliofibularis tubercle is preserved. Its medial aspect is flattened distally, becoming slightly concave proximally ( Fig. 3b ). The shaft is relatively uniform throughout its length, exhibiting a slight craniocaudal expansion proximally. Preserved portions of the pes include the distal end of the third metatarsal and a badly damaged portion of the distal articulation of metatarsal II or IV, as well as pedal phalanges II-1, III-2 and IV-3 ( Fig. 3f,g ). Collateral ligament fossae are deep and surrounded by a broader secondary depression as in other allosauroids ( Fig. 3g ), unlike the shallow fossae of megalosauroids. Phylogenetic analysis We recover Siats as a carcharodontosaurian allosaurian ( Fig. 4 ) based largely on the extent and nature of pneumatic features, which include pleurocoels on dorsal and likely also on sacral vertebral centra, and honeycombed or ‘camellate’ interior pneumaticity, as well as alariform morphology of dorsal hyposphens and peg and socket ilio-ischial articulation. The presence of tab-like lateral extensions on the dorsal postzygapophyses ( Fig. 2e ) and externally piercing pneumaticity of the prezygapophyses ( Fig. 2b ), prominent centrodiapophyseal laminae on caudal neural arches ( Fig. 2h ), and presence of a preacetabular cuppedicus shelf ( Fig. 3a ) posit Siats as a member of the subclade Neovenatoridae. A placement within the subclade Megaraptora is supported by pronounced centrodiapophyseal laminae bracketed by deep infradiapophyseal fossa on the caudal neural arches ( Fig. 3h ), which we interpret as homologous with the condition observed in Aerosteon [26] and Megaraptor [25] . A Bremer support value of >5 indicates strong support for a monophyletic Neovenatoridae including Siats ( Fig. 4b ). Siats remains labile within Megaraptora, largely due to lack of skeletal overlap between select taxa, but combinable component (= semi-strict) consensus trees posit Chilantaisaurus as sister taxon to all other megaraptorans including Siats ( Fig. 4b ). Unresolved ancestral relationships between Asian, Australian and South American megaraptorans persist, contributing to an ambiguous paleobiogeographical history of the clade. 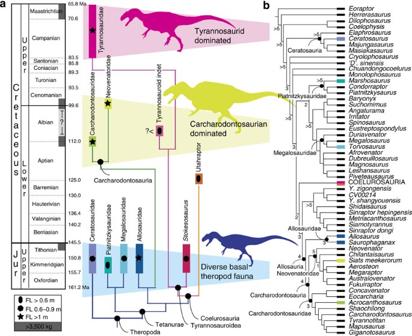Figure 4: Evolutionary relationships of apex predators in the Late Jurassic and Cretaceous of North America. Apex predator role defined as largest predators per time bin, generally estimated as species with a femur length >1 m15; (a) trifaunal characterization of predator guilds with unique taxonomic and mass compositions: a diverse, mixed mass, Late Jurassic predator assemblage, mid-Cretaceous gigantic carcharodontosaurian dominated fauna and terminal large-bodied to gigantic tyrannosaurid guild. Grey boxes on timescale to left indicate spans when apex predators achieved gigantism, topping estimates of 3,500 kg30. Chronostratigraphic occurrences follow30; (b) combinable component consensus tree showing taxonomy and relationships of North American predators during this interval andS. meekerorumposited as a megaraptoran neovenatorid. Numbers at nodes denote Bremer support values. Taxon colours consistent between partsaandb. Ma equals million years ago. Figure 4: Evolutionary relationships of apex predators in the Late Jurassic and Cretaceous of North America. Apex predator role defined as largest predators per time bin, generally estimated as species with a femur length >1 m [15] ; ( a ) trifaunal characterization of predator guilds with unique taxonomic and mass compositions: a diverse, mixed mass, Late Jurassic predator assemblage, mid-Cretaceous gigantic carcharodontosaurian dominated fauna and terminal large-bodied to gigantic tyrannosaurid guild. Grey boxes on timescale to left indicate spans when apex predators achieved gigantism, topping estimates of 3,500 kg [30] . Chronostratigraphic occurrences follow [30] ; ( b ) combinable component consensus tree showing taxonomy and relationships of North American predators during this interval and S. meekerorum posited as a megaraptoran neovenatorid. Numbers at nodes denote Bremer support values. Taxon colours consistent between parts a and b . Ma equals million years ago. Full size image Extensive apex predator guild restructuring in the Early Cretaceous of western North America is evidenced by a shift from well known Late Jurassic assemblages consisting of multiple clades of medium to large-bodied theropods towards terminal Cretaceous ecosystems dominated exclusively by large (2,000–5,000 kg) to gigantic (>5,000 kg) tyrannosaurids [4] , [28] ( Fig. 4a ). However, the pace and nature of this transformation has been largely unknown due to a near 70 million year gap in the apex predator record of western North America. Discovery of Siats , a gigantic megaraptoran neovenatorid, in mid-Cretaceous ecosystems, together with new phylogenetic interpretations positing Acrocanthosaurus in a more derived position within Carcharodontosauridae [14] , [19] , [29] , [30] indicate that apex predator guilds of that time were composed neither of relic Jurassic theropod clades nor by early replacement by tyrannosaurids, and that two-step depictions of predator communities are insufficient to describe theropod guild evolution during this interval. Rather, these data indicate that mid-Cretaceous theropod assemblages were taxonomically unique from both prior and subsequent faunas in being composed largely of derived carcharodontosaurians (with subsidiary roles occupied by one or more clades of medium-bodied coelurosaurian) and that, minimally, a trifold characterization of apex predator guild occupancy mirroring the pattern observed in Asia [11] , [14] is required ( Fig. 4a ). Persistence of carcharodontosaurian theropods into the Late Cretaceous has recently been invoked as an explanation for the delayed ascent of tyrannosaurids as apex predators in Asian ecosystems [14] , [15] . Siats not only provides the first evidence for megaraptoran allosauroids in North America, but also demonstrates that carcharodontosaurians continued to occupy apex guilds on the continent into the Late Cretaceous, possibly constraining tyrannosauroid size evolution via competitive exclusion throughout the mid-Cretaceous [11] , [19] . This suggests that competitive exclusion of tyrannosauroids from keystone predator niches by allosauroids can be extrapolated across much of Laurasia. More importantly, it offers a direct test of this hypothesis, because the Mussentuchit faunal assemblage preserves evidence of ecological sympatry between colossal allosauroids and diminutive tyrannosauroids [31] , [32] . Temporal overlap between allosauroids and putative tyrannosauroids in Gondwana is noted from a single locality in southern Australia [33] , although these are based on more fragmentary remains. By contrast, although ghost lineages subtended by these clades suggest such evidence may be forthcoming, carcharodontosaurians are not yet definitively documented from the same Asian rock units as tyrannosauroids. The presence of Siats in Cenomanian ecosystems reduces the temporal gap between the decline of carcharodontosaurians and rise of tyrannosauroids as apex predators in western North America to 15 million years marked by a sea level highstand and a poor terrestrial record [11] , and within 7 million years of the turnover in Asia. To date, carcharodontosaurians are not known to have survived past the Turonian (~92 Ma) on Laurasian landmasses [11] , [30] and also decline in South America over the same timeframe [34] , [35] ( Fig. 5a ). The actual timing of allosauroid extirpation in Asiamerica is as of yet unclear, due to the paucity of Turonian through Santonian continental deposits ( Fig. 5a ) but it clearly postdates the Cenomanian–Turonian boundary. With the discovery of Siats , Megaraptora is notable for representing a cosmopolitan clade that inhabited most major continents despite advanced stages of continental rifting in the mid-Cretaceous [36] . 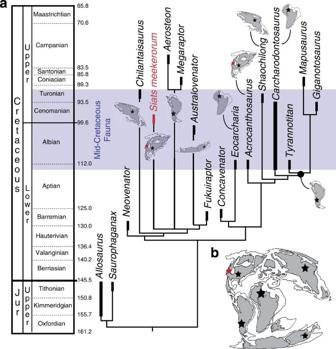Figure 5: Distribution of Carcharodontosauria in time and space. (a) Combinable component consensus tree showing chronostratigraphic distribution of Allosauria; (b) mid-Cretaceous (Aptian-Cenomanian) paleobiogeographic map of Carcharodontosauria, illustrating the former western North American gap filled by discovery ofSiats. Previously known generalized areas denoted with black stars, newly described distribution in western North America marked with red star. Map adapted from ref.69with permission from Elsevier. Figure 5: Distribution of Carcharodontosauria in time and space. ( a ) Combinable component consensus tree showing chronostratigraphic distribution of Allosauria; ( b ) mid-Cretaceous (Aptian-Cenomanian) paleobiogeographic map of Carcharodontosauria, illustrating the former western North American gap filled by discovery of Siats . Previously known generalized areas denoted with black stars, newly described distribution in western North America marked with red star. Map adapted from ref. 69 with permission from Elsevier. Full size image Just as the biodiversity of mid-Cretaceous North American apex predators differs considerably from that observed in prior and subsequent time bins, so too does its biogeographic history. Predator guilds of the Late Jurassic include a variety of large theropod genera shared with other continents [15] , whereas, latest Cretaceous megapredator diversity exhibits largely endemic biogeographic patterns with abelisaurids dominating Gondwanan continents, tyrannosaurids ruling Asiamerican ecosystems, and their respective distributions constrained by the coupling of continental isolation [11] , [15] , [37] , [38] , [39] and high sea levels [40] . Therefore, apex predator faunas, at least in North America, appear to follow a trend from high phylogenetic diversity and low endemism to the opposite extreme of low diversity and pronounced endemism. North American mid-Cretaceous assemblages represent a transition between these extremes in that they are currently characterized by low diversity (although this may be related to sampling bias) and low to moderate endemism, with sister taxa occurring on at least two other continents [41] . A similar pattern is also evident in abelisaurid [38] and spinosaurid [42] theropods. Such low levels of theropod endemicity are closer to those observed in Early Jurassic Pangaean theropod faunas, than to the more taxonomically depauperate latest Cretaceous faunas. With regard to Carcharodontosauria, basal most and/or oldest members of both its constituent subclades (for example, Neovenator , Chilantaisaurus , Siats , Concavenator , Acrocanthosaurus , Shaochilong , Veterupristisaurus and Neovenatoridae indet from Australia) are distributed across both Laurasian and Gondwanan landmasses [33] , [43] ( Fig. 5 ) supporting hypotheses of near global distribution of theropod clades until the latest Cretaceous that stem from Jurassic origins [11] , [43] , [44] . Although, the identification of a derived neoventatorid (that is, Megaraptora), and a derived carcharodontosaurid ( Acrocanthosaurus [30] ) in mid-Cretaceous ecosystems of North America ( Fig. 5b ) is consistent with growing evidence suggesting that the majority of theropod clades had global or near global distributions until the latest Cretaceous [11] , [33] , [44] it is also consistent with biogeographic hypotheses involving continental scale dispersal across portions of Laurasia during this interval. Phylogenetically informed biodiversity data from a range of terrestrial vertebrates inhabiting western North America have spurred hypotheses of local extirpation and dispersal that may correlate with subaerial exposure of an Asian-North American land bridge in the Aptian/Albian [18] , [32] , [45] , [46] , [47] – a hypothesis dubbed EKLInE [32] . The sum of these occurrences largely derive from the early Late Cretaceous Mussentuchit Member of the Cedar Mountain Formation and the late Early Cretaceous Cloverly Formation and suggest minimal initiation by the Albian with the possibility that dispersal spanned the Early-Late Cretaceous boundary. Chronostratigraphic and evolutionary relationships of mammals [48] , squamates [49] , trionychoid turtles [50] , ornithischian dinosaurs [31] , [32] , [47] , [51] and coelurosaurian theropods including derived tyrannosauroids [31] from these formations provide intriguing if sometimes tentative support for such interchange. However, unlike microfaunal components, for which we have rich fossil data [18] , [49] many of the dinosaurian records are restricted to fragmentary skeletal remains that have not been subjected to rigorous biogeographic analysis or are substantiated by robust data (see for example, ref. 52 ). Others, such as the appearance of therizinosaurids in the Turonian of North America [53] and relationships among iguanodontians [51] , which are known from more complete skeletons, are more compelling, yet fewer in number. Although Siats fills a critical gap in the biogeographic history of Early to mid-Cretaceous theropods, the poor fossil record of the group globally [11] , [29] , [34] , [43] , [44] , various possible resolutions of Megaraptora in our analyses, and long ghost lineages subtended by most megaraptoran species continue to permit both global distribution and interchange biogeographic scenarios with equal likelihood. Increased resolution of neovenatorid relationships and increased sampling of Early Cretaceous theropods around the globe will be necessary to test ancestral geographic origins for Siats and other carcharodontosaurians. Size class estimation We interpolated an estimate for the femoral length (FL) of Siats , a widely used proxy for body size in dinosaurs [54] , [55] , [56] , from regressions against diaphyseal measurements of the fibula [28] . The fibula exhibits a phylogenetic trend towards diaphyseal reduction across theropod evolution, which we accounted for by employing Phylogenetic Independent Contrasts [57] to find the regressions and their confidence intervals. Phylogenetically corrected predictions of FL ranged from 1,166 to 1,410 mm depending on which fibular metric was employed. We conservatively employ the lower estimate and note that these data are extrapolated from an immature individual, further reducing potential inflation of our estimated FL for this taxon. An estimated FL of 1,166 mm approximates the 1,190 mm reported for the closely related Chilantaisaurus from China, and thus Siats is one of the largest megaraptorans recorded. Our size estimates also compare well with the 1,266 mm observed in the stratigraphically older carcharodontosaurid Acrocanthosaurus from the Albian Cloverly and Trinity formations, and also the latest Jurassic allosauroid Saurophaganax , which has an 1,135 mm long femur. Moreover, Siats was by far larger than the four or more other theropod taxa documented in the Mussentuchit [32] , and well above the one ton estimate employed by previous authors to define apex predators [15] . Size class estimates for Jurassic and Cretaceous theropods ( Table 2 ) were generated using known or interpolated FL and the theropod specific equation relating body mass to FL [28] . These values were used to place large-bodied theropod species into generalized mass bins and identify time spans where apex predators achieved relative gigantism (>3,500 kg). We recognize that mass extrapolation adds additional uncertainty to size estimates over FL alone, specifically among clades with variable bauplans [58] . However, we do not use mass estimates as point values here and binning protocol minimizes point value error. This practice follows(15) in using binned mass values (>1 metric ton) as definitional modifiers for apex predator species. Table 2 Estimated size class and body mass for theropods inhabiting the Late Jurassic through Late Cretaceous in western North America. Full size table Some taxa in this study lack a preserved femur. In these cases, we used the principles of patristic distance and allometric scaling to generate reasonable FL estimates allowing us to bin taxa by gross size class. Torvosaurus and Marshosaurus lack preserved femora, therefore we estimated FL in these taxa using femur/tibia ratios derived from the relatively complete skeletons of other tetanuran theropods. For Torvosaurus [59] (TL=725 mm) we calculated a FL range of 754–783 and a body mass range of 961–1086, kg using femur/tibia ratios derived from Eustreptospondylus [60] (OUMNH J.13558: FL= 498 mm, TL=479 mm) and Megalosaurus bucklandii [61] (OUM J13561, FL=810, TL=650). We based hind limb ratios for Marshosaurus on the similar-sized megalosauroid Eustreptospondylus [60] whose femur length (498 mm) to ilium (365 mm) ratio is 1.36. This yielded a minimum FL for Marshosaurus (UMNH VP 6373) of 544 mm based on an estimated ilium that is a minimum of 400 mm long. Minimum body mass estimate for Marshosaurus is likely within the range of 300–400 kg. A femur length estimate of 520 mm for Utahraptor [62] was interpolated based on the hind limb ratio of the similarly sized dromaeosaurid Achillobator [63] (FR.MNUFR-15) (tibia length 490.4 mm, femur length 505 mm, ratio). This value yields a body mass estimate for Utahraptor of ~290 kg. Phylogenetic protocol We examined the evolutionary relationships of Siats by inclusion in a recent, comprehensive analysis of tetanuran theropods [30] , including 61 theropods (48 tetanurans) and 355 characters ( Supplementary Note 1 and Supplementary Data 1 ). We added new characters, modified select character scores and excluded characters in the base matrix ( Supplementary Note 1 and Supplementary Data 1 ). Character parameters were set following Carrano et al. [30] Data coding, character tracing and tree manipulation/visualization were carried out using Mesquite ver. 2.75 (ref. 64 ). Phylogenetic analyses were executed in the program TNT [65] . We conducted heuristic searches on Wagner trees using TBR (tree bisection–reconnection) branch-swapping with 1,000 random addition sequences holding 10 trees per replicate continuing subsequent TBR swapping on all stored minimum length trees (4,860 most parsimonious trees, TL=1,039). We assessed results using strict, semi-strict and reduced consensus methods and Bremer support values [66] . Ambiguous nodes were collapsed following Rule 1 of Coddington and Scharff [67] . Maximum agreement subtrees [68] were calculated in TNT and used to identify labile taxa and common topology among all MPTs. We followed Carrano et al. [30] in ad hoc pruning of Poekilopleuron , Streptospondylus and Xuanhanosaurus from consensus trees, although this did not change topology within Allosauria. A recent phylogenetic study posited megaraptorans as basal tyrannosauroids [69] . We did not test Siats by inclusion in this dataset, but note that of the three of the features listed as synapomorphies of these clades that can be coded on Siats , two are absent (constriction of fibular shaft and brevis shelf hidden in lateral view). This suggests that the inclusion of Siats might cause re-optimization of some characters supporting this novel topology. Nomenclatural act This published work and the nomenclatural acts it contains have been registered in ZooBank, the proposed online registration system for the International Code of Zoological Nomenclature (ICZN). The ZooBank LSIDs (Life Science Identifiers) can be resolved and the associated information viewed through any standard web browser by appending the LSID to the prefix ‘ http://zoobank.org/ ’. The LSID for this publication is urn:lsid:zoobank.org:pub:D17340F3-CE3A-43D9-A4F8-403F8FF18D20. How to cite this article: Zanno, L. E. and Makovicky, P. J. Neovenatorid theropods are apex predators in the Late Cretaceous of North America. Nat. Commun. 4:2827 doi: 10.1038/ncomms3827 (2013).